Expanded graphite as superior anode for sodium-ion batteries Graphite, as the most common anode for commercial Li-ion batteries, has been reported to have a very low capacity when used as a Na-ion battery anode. It is well known that electrochemical insertion of Na + into graphite is significantly hindered by the insufficient interlayer spacing. Here we report expanded graphite as a Na-ion battery anode. Prepared through a process of oxidation and partial reduction on graphite, expanded graphite has an enlarged interlayer lattice distance of 4.3 Å yet retains an analogous long-range-ordered layered structure to graphite. In situ transmission electron microscopy has demonstrated that the Na-ion can be reversibly inserted into and extracted from expanded graphite. Galvanostatic studies show that expanded graphite can deliver a high reversible capacity of 284 mAh g −1 at a current density of 20 mA g −1 , maintain a capacity of 184 mAh g −1 at 100 mA g −1 , and retain 73.92% of its capacity after 2,000 cycles. The Li-ion battery (LIB) industry has been continuously expanding over the last three decades, mostly because of the steadily increasing demands of a growing market for portable electronic devices. However, as demand emerges for hybrid and electric vehicles, and as emphasis shifts to the power grid and other large-scale applications, the limits of the natural abundance and uneven global distribution of lithium-containing precursors present unavoidable challenges to industry. For such large-scale applications, a low-cost and sustainable supply-chain is critical. As an alternative, Na-ion batteries (NIBs) have recently drawn significant attention because, unlike Li, Na is a ubiquitous and earth-abundant element. NIBs were originally developed in the late 1980s, in approximately the same time period as LIBs [1] , [2] , [3] , and the demand for large-scale energy storage for grid applications has recently revived the interest. Most of the recent research on NIB electrode materials has focused mainly on cathodes, but here we concentrate instead on a possible new anode material. Since Li and Na share common properties as alkali metals, it is sometimes assumed to be convenient to transfer the insights gained from the science of LIBs to NIBs. However, Na + has a larger radius than Li + , which directly affects the mass transport and storage in the electrochemical process. It makes many of the superior LIB anode materials, such as graphite, unsuitable for NIBs. Graphite, as the most common anode for commercial LIBs, has a long-range-ordered layered structure, and Li + can readily electrochemically intercalate between the graphite layers. The intercalated material has a high theoretical reversible capability of 372 mAh g −1 and long cycle life. However, the electrochemical sodiation/desodiation capacity of graphite is <35 mAh g −1 (refs 4 , 5 ). As demonstrated by recent theoretical calculations, the interlayer distance of graphite (~0.34 nm) is too small to accommodate the large Na + ion ( Fig. 1a ), and a minimum interlayer distance of 0.37 nm is believed to be required for Na + insertion [6] . 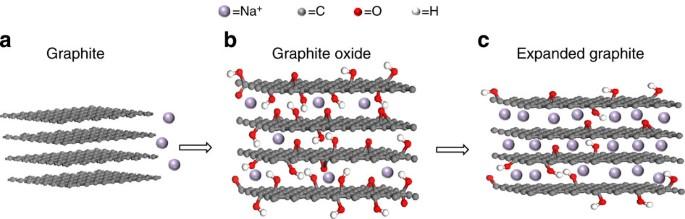Figure 1: Schematic illustration of sodium storage in graphite-based materials. (a) Na+cannot be electrochemically intercalated into graphite because of the small interlayer spacing. (b) Electrochemical intercalation of Na+into GO is enabled by the enlarged interlayer distance because of oxidation. However, the intercalation is limited by steric hindering from large amounts of oxygen-containing groups. (c) A significant amount of Na+can be electrochemically intercalated into EG owing to suitable interlayer distance and reduced oxygen-containing groups in the interlayers. Figure 1: Schematic illustration of sodium storage in graphite-based materials. ( a ) Na + cannot be electrochemically intercalated into graphite because of the small interlayer spacing. ( b ) Electrochemical intercalation of Na + into GO is enabled by the enlarged interlayer distance because of oxidation. However, the intercalation is limited by steric hindering from large amounts of oxygen-containing groups. ( c ) A significant amount of Na + can be electrochemically intercalated into EG owing to suitable interlayer distance and reduced oxygen-containing groups in the interlayers. Full size image A variety of carbon materials, such as carbon with different structures (soft carbons [5] and hard carbons [5] , [7] , [8] ), different compositions (hydrogen-contained carbons [5] ) and different morphologies (carbon nanotubes [6] , porous carbons [9] , hollow carbon nanoparticles [10] and reduced graphene oxides [11] ), have been investigated as anodes for NIB in previous studies. Most of these carbon-based materials consist of few-layer-stacked graphite nanocrystallites with large interlayer distances in the range of 0.37–0.40 nm (ref. 6 ). These localized nanocrystallites leave many disordered nanovoids within the materials [5] , [6] , [9] , [10] , [11] , [12] , and it is believed that the Na + ions can reversibly insert into the graphite nanocrystallites and the nanovoids in these carbon materials. Na + insertion in nanocrystallite usually occurs in a wide potential range from 1.5 to 0.1 V (versus Na/Na + ), whereas the Na + filling into nanovoids happens in a low and narrow potential range of 0.1–0.0 V (versus Na/Na + ) [5] , [6] , [9] , [10] , [11] , [12] . In these two mechanisms, the interlayer insertion reaction would be preferred, as the pore-filling reaction occurs only at low potentials, where it can be accompanied by Na plating during fast charging, causing Na loss and, more severely, battery failure due to electrical shorting. Certain conclusions can be drawn from these studies, and it is apparent that materials with long-range-ordered layered structures, larger interlayer distances and low porosity are desired. Here we report expanded graphite (EG) as a superior NIB anode material. EG is a graphite-derived material formed by a two-step oxidation-reduction process that retains the long-range-ordered layered structure of graphite, yielding a generally large interlayer distance (>0.34 nm; Fig. 1b,c ). These features provide favourable conditions for electrochemical intercalation of Na + ions. Moreover, the interlayer spacing of EG can be manipulated by controlled oxidation and reduction processing, which positions EG as a promising anode material for NIBs. We report here that Na + indeed can reversibly insert into and extract from the EG, with an interlayer distance of 0.43 nm. The sodiation- and desodiation-induced microstructure changes of EG are dynamically captured during real-time imaging at the atomic scale using in situ high-resolution transmission electron microscopy (HRTEM). Electrochemical tests show that the EG can provide a high reversible capacity of 284 mAh g −1 at a current density of 20 mA g −1 ; 184 mAh g −1 at a current density of 100 mA g −1 ; and retain 73.92% of the capacity after 2,000 cycles (loss 0.037% per cycle). Along with the mature and low-cost synthesis technique of graphite anodes for LIBs, EG could be a very promising anode material for the NIBs industry in the near future. Material and structural design EG was synthesized by oxidizing pristine graphite (PG) to become graphite oxide (GO) using modified Hummer’s method [13] and followed by a partial reducing process of GO. The modified Hummer’s method is well known as an oxidization method to form GO in the graphene synthesis technique [11] . In a typical graphene synthesis procedure, the resulting GO is sonicated before (or after) the reduction reaction to peel off the functionalized graphene layers from graphite and acquire single-layer or few-layer graphenes. In our synthesis, we intentionally omitted the sonication step to avoid the damage caused by sonication and maintain the long-range-ordered layered structure. More experimental details are provided in Methods section. The crystal structures of PG, GO and two EG samples (EG-1 h and EG-5 h with 1 h/5 h denoting the thermal reduction period applied on GO to obtain the sample) were characterized using powder X-ray diffraction (XRD; Supplementary Fig. 1 ). For the purpose of systematically analysing the reduction time effect, GO was considered as EG-0 h to compare with EG samples (EG-1 h and EG-5 h). PG exhibits a sharp peak at 2θ ~26.6° ( Supplementary Fig. 1 ), which corresponds to the diffraction of (002) plane with an interlayer distance of 3.36 Å (~0.34 nm) (refs 14 , 15 ). Upon oxidation, the inserted oxygen-containing groups will attach to both sides of the single graphene plane, causing distortion of the interlayer structure [16] , [17] . The diffraction peak of GO shifts to 2θ ~13.0°, which indicates an enlarged inter-planar distance. After thermal reduction for 1 h, the diffraction peak of EG-1 h shifts back to 2θ ~23.0°, yet is still smaller than that in graphite (~26.6°), exhibiting a graphite-like structure with a larger inter-planar distance. As thermal reduction time increases to 5 h, the diffraction peak of EG-5 h shifts to 2θ ~25.3°, indicating a shrinkage of interlayer distance compared with EG-1 h. The surface areas of PG, GO and EG samples were characterized by using N 2 gas adsorption–desorption. The Brunauer–Emmett–Teller (BET) surface areas are measured to be 13.52 m 2 g −1 for PG, 64.89 m 2 g −1 for GO, 30.22 m 2 g −1 for EG-1 h and 34.70 m 2 g −1 for EG-5 h. Both EG samples reveal a low surface area, which is much smaller than that of typical graphene/graphene oxide prepared through Hummer’s method [18] , indicating low exfoliation degree and good graphite-like stack morphology retention. On the other hand, the low surface area of EGs also implies that only a small amount of pores are introduced during oxidation and thermal reduction process. Different from graphite, the N 2 adsorption–desorption isotherm profiles of GO, EG-1 h and EG-5 h exhibit no limiting adsorption at high P/P 0 ( Supplementary Fig. 2a ), revealing a typical character of plate-like particle with slit-shaped pores [19] . The specific surface area of PG used in this study is three times higher than that of previously reported graphite [20] , and is similar to that of the hard carbon (SX114i19 in ref. 21 ). The EGs’ surface areas are similar to the hard carbon (SX114i5 in ref. 21 ) reported by Dahn and group [21] . The tap densities for PG, GO, EG-1 h and 5 h samples were measured to be 0.72, 4.38, 2.38 and 1.88 g cm −3 ( Supplementary Fig. 2b ). The tap densities of EG samples are higher than that of most of reported soft carbons (~0.66–1.26 g cm −3 ; (ref. 22 ) and hard carbon (~0.50–0.81 g cm −3 ; (refs 22 , 23 ), whereas the PG’s tap density is similar to the hard carbon [21] . The EG samples were observed to be more condensed than the reported carbon material used in LIB [21] . The graphitization degree of PG, GO and EG materials was determined by Raman spectroscopy. All samples exhibit typical D band (centred at ~1,360 cm −1 ) and G band (centred at~1,585 cm −1 ) for carbon material [24] . The D band corresponds to the disordered carbon, whereas the G band represents the typical signal for graphite-like morphology in carbon material. The I D / I G intensity ratios for PG, GO, EG-1 h and EG-5 h are 0.22, 0.86, 0.88 and 0.97 ( Supplementary Fig. 2c ), indicating that EGs partially maintain the graphitic character. The electronic conductivities of PG, GO, EG-1 h and EG-5 h were measured to be 461.47, 87.65, 322.62 and 363.40 S cm −1 , respectively ( Supplementary Fig. 2d ). Both EG samples show much better conductivity than GO (EG-0 h) because of the removal of oxygen-containing groups during thermal reduction. The structures of PG, GO and EGs were further characterized by TEM. 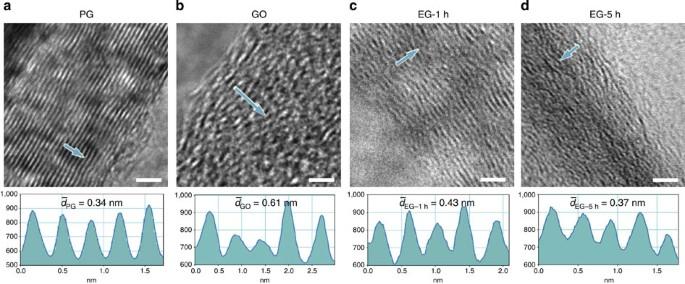Figure 2: High-resolution TEM analysis of PG, GO and EG. High-resolution TEM images showing cross-sectional layered structures for (a) PG, (b) GO, (c) EG-1 h and (d) EG-5 h. Scale bars, 2 nm. Contrast profiles along the arrows indicate interlayer spacings of corresponding samples. Figure 2 shows HRTEM images of the cross-sectional view for PG, GO, EG-1 h and EG-5 h, in which the layered structures of these specimens are well resolved by the alternating bright and dark contrast. The PG displays well-defined layers of long-range order stacking parallel to each other ( Fig. 2a ). After oxidation, such long-range order is disrupted by massive intercalation of oxygen in the graphite interlayer, forming a more disordered pattern with only localized short-range ordering, as shown in Fig. 2b . However, after partial reduction, the material recovers toward a well-organized morphology, while preserving expanded interlayer distances and the long-range channels suitable for Na ions transport, as shown in Fig. 2c,d . In addition, the progressive change in interlayer distance is also clearly apparent. The contrast line profiles across five stacking layers at representative locations, indicated by the arrows, are plotted under the corresponding images. The average interlayer spacings are measured to be ~0.34 nm for PG, 0.61 nm for GO, 0.43 nm for EG-1 h and 0.37 nm for EG-5 h. It is obvious that the distance between PG layers is expanded after the oxidation reactions because of the insertion of oxygen-containing groups, and that it still retains larger than PG after reduction treatments. Figure 2: High-resolution TEM analysis of PG, GO and EG. High-resolution TEM images showing cross-sectional layered structures for ( a ) PG, ( b ) GO, ( c ) EG-1 h and ( d ) EG-5 h. Scale bars, 2 nm. Contrast profiles along the arrows indicate interlayer spacings of corresponding samples. Full size image Nature and content of oxygen-containing groups in the interlayer From above XRD and HRTEM results, it is clear that the interlayer distances of PG, GO and EGs are related to the nature and content of oxygen-containing groups in the interlayer. So, the nature and amount of these oxygen-containing groups in PG, GO and EG samples (EG-1 h and EG-5 h) were investigated using X-ray photoelectron spectroscopy (XPS), and the results are shown in Fig. 3a–d , where C 1 s peak presents at ~284.8 eV and O 1 s peak presents at ~533.6 eV. 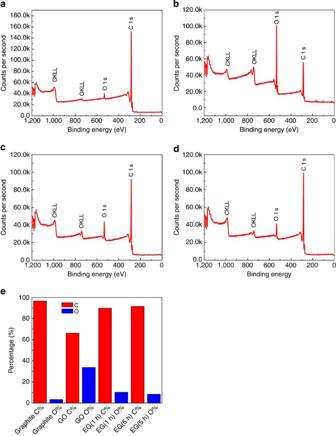Figure 3: XPS investigation of the oxygen content. Wide-range XPS spectra of (a) graphite, (b) GO, (c) EG-1 h (d) EG-5 h and (e) percentage of C and O element ratio in different samples. Figure 3e illustrates the C/O ratio calculated from the intensity of C 1 s and O 1 s peaks for different samples. PG contains a very small amount of oxygen (3.56%) ( Fig. 3a ). Upon oxidation, the intensity of O 1 s peak increases significantly ( Fig. 3b ) and the oxygen component reaches to 33.82%, indicating a high oxidation state. After 1 h thermal reduction in argon (Ar), the oxygen content of EG-1 h sample reduces to ~10% ( Fig. 3c ), which is much less than that in GO, but it is still three times higher than that in PG. The residual 10% oxygen-containing groups maintain the interlayer distance at ~0.43 nm ( Fig. 3c ). As the reduction time increases from 1 to 5 h, the oxygen content further drops to 8% in EG-5 h. The 2% decrease in O component was attributed to further loss of functional groups between graphene layers, resulting in some shrinkage of the interlayer distance, as evidenced by the HRTEM results in Fig. 2d . Figure 3: XPS investigation of the oxygen content. Wide-range XPS spectra of ( a ) graphite, ( b ) GO, ( c ) EG-1 h ( d ) EG-5 h and ( e ) percentage of C and O element ratio in different samples. Full size image The nature of oxygen-containing functional groups was further analysed by the high-resolution C 1 s scans ( Supplementary Fig. 3 ). The minor O component in PG exists in the form of C–OH or C–O–C groups ( Supplementary Fig. 3a ), whereas the O content in GO mainly exists as C–OH, C–O–C and C=O components ( Supplementary Fig. 3b ). After thermal reduction, most of the oxygen-containing groups in GO are removed. A small amount of residual O in the interlayer exist as C–OH/C–O–C and C=O groups in EG-1 h and EG-5 h ( Supplementary Fig. 3c,d ). The structure evolution along oxygen-containing groups amount change was further investigated by magic-angle-spinning nuclear magnetic resonance (MAS-NMR) experiment. In the 13 C spectrum of GO ( Fig. 4a ), three major peaks at 131, 69 and 61 p.p.m. evidence the occurring of the oxidization that is consistent to the previous study [25] , [26] . The weak peaks at ~165 and ~190 p.p.m. (indicated by blue arrows) can be assigned to –CO 2 – and C=O [27] , consistent with the XPS measurements. The EG-1 h and EG-5 h samples show a single broader major peak at 117 p.p.m. ( Fig. 4b ) and 116 p.p.m. ( Fig. 4c ) with another broad shoulder peak at ~170 p.p.m. The observed 13 C shifts are consistent with those for sp 2 carbons without oxidized sites (~120 p.p.m.) such as graphene or graphite, suggesting the restoration of sp 2 conjugation network. The change in the 13 C shift position for the sp 2 species from ~130 p.p.m. in GO to ~120 p.p.m. in EG reflects the removal of electron-withdrawing oxygen-containing groups by the reduction. No noticeable peaks were observed either at 60 or 70 p.p.m., although a weak peak for the C–OH group may overlap with a tail of the sp 2 carbons at 120 p.p.m. The results suggest that thermal reduction for 1 h is sufficient to restore the sp 2 network in the EG sample. Based on the integral intensities of the spectra at 40–80 p.p.m. region in Fig. 4b,c , these oxidized species should constitute ~3–8% of the carbon. This portion of the carbon can be attributed to the C–OH or epoxide from graphene plane that is highly related to the interlayer spacing. The broad shoulder peak at ~170 p.p.m. may be attributed minor species (such as C=O and –CO 2 H species) that could be found around the edges/defects. Minor discrepancies from the XRD results may be attributed to the oxygen species at the edges/defects. 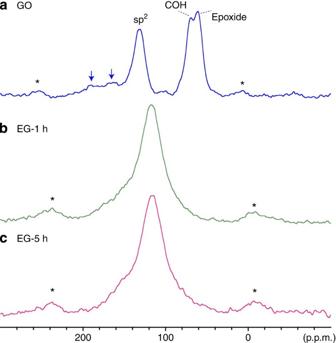Figure 4: Solid-state NMR study. 1D13C MAS solid-state NMR spectra of (a) GO, (b) EG-1 h and (c) EG-5 h. All the spectra were obtained at a13C NMR frequency of 125.78 MHz with 15 kHz MAS for the samples of (a) 33 mg, (b) 38 mg, (c) 45 mg. The13C MAS spectra were obtained with direct13C excitation by a π/2-pulse followed by a rotor-synchronous echo. The peaks marked by * denote spinning sidebands. The recycle delay was 2 s, and the experimental times were (a) 3 h and (b,c) 7 h. A Lorentz broadening of 300 Hz was applied to improve the signal-to-noise ratios.13C T1values of the samples were found to be 0.5–0.6 s. The13C π/2-pulse widths are (a) 3.65 μs and (b,c) 5.75 μs. Figure 4: Solid-state NMR study. 1D 13 C MAS solid-state NMR spectra of ( a ) GO, ( b ) EG-1 h and ( c ) EG-5 h. All the spectra were obtained at a 13 C NMR frequency of 125.78 MHz with 15 kHz MAS for the samples of ( a ) 33 mg, ( b ) 38 mg, ( c ) 45 mg. The 13 C MAS spectra were obtained with direct 13 C excitation by a π/2-pulse followed by a rotor-synchronous echo. The peaks marked by * denote spinning sidebands. The recycle delay was 2 s, and the experimental times were ( a ) 3 h and ( b , c ) 7 h. A Lorentz broadening of 300 Hz was applied to improve the signal-to-noise ratios. 13 C T 1 values of the samples were found to be 0.5–0.6 s. The 13 C π/2-pulse widths are ( a ) 3.65 μs and ( b , c ) 5.75 μs. Full size image To identify C–OH groups and other 1 H-containing species in the GO and EG samples, 13 C– 1 H dipolar dephasing experiments were performed by using a 13 C– 1 H rotational echo double resonance (REDOR) pulse sequence. It is notable that for GO sample, the signal for C–OH was mildly dephased ( Supplementary Fig. 4 ). The difference between non-dephased spectrum ( Supplementary Fig. 4a ) and dephased spectrum ( Supplementary Fig. 4b ) clearly shows that the signal intensities for the C–OH and epoxide groups are reduced by about 20% and 13%, respectively, whereas the intensity for the sp 2 group is reduced by only 6%. The strongest dephasing is a direct evidence of the existent of massive oxygen-containing species, especially the C–OH, in GO. This approach is adopted to analyse EG-1 h and EG-5 h. Supplementary Fig. 5 shows 13 C MAS spectra of EG-1 h ( Supplementary Fig. 5a–c ) and EG-5 h ( Supplementary Fig. 5d–f ) without and with 13 C– 1 H dipolar dephasing by 13 C– 1 H REDOR, together with corresponding difference spectra ( Supplementary Fig. 5c,f ). For the both samples, no notable selective dephasing was observed unlike the above-mentioned experiment for GO. Rather, the peaks corresponding to sp 2 group at ~120 p.p.m. were uniformly dephased for EG-1 h ( Supplementary Fig. 5c ) and EG-5 h ( Supplementary Fig. 5f ) by 12% and 8%, respectively. It is noteworthy that the signal reduction is higher than that was observed for sp 2 species in GO. The results indicate that the surface of the restored graphene sheets in EG can be covered by hydrogen-containing species, and these species may be, in part, responsible for expanded interlayer distances. Indeed, that EG-5 h shows a lower dephasing than EG-1 h, which is consistent with the observed smaller interlayer distance for EG-5 h. Effect of oxygen content on sodium storage capacity Theoretical calculations have revealed that when the interlayer spacing increases to ~0.37 nm, the energy barrier for Na + insertion drops to 0.053 eV (ref. 6 ). This calculation suggests that it is thermodynamically feasible to electrochemically insert Na + into EG-1 h. Although a large interlayer distance is desired for Na + insertion, too many oxygen-containing groups between graphene layers could reduce the available positions for Na + and slow the Na + transport. The amount of remaining oxygen-containing groups in the interlayer of EG should in principle be optimized to maintain the sufficient interlayer distance and maximize possible positions for Na-ion storage. The effects of oxygen content on sodiation/desodiation capacity were investigated using galvanostatic charge/discharge at a current density of 20 mA g −1 . The charge and discharge curves of PG, GO, EG-1 h and EG-5 h at the second cycles are presented in Fig. 5a . Retarded by the small interlayer spacing, PG has a negligible sodium storage capacity of ~13 mAh g −1 , which is widely known and has been reported previously [28] . Oxidation of graphite increases the interlayer distance from 0.34 to 0.61 nm, allowing Na + intercalation into interlayer of GO. The GO shows monotonic voltage curves during the whole sodiation–desodiaton process with an increased capacity of ~156 mAh g −1 . However, 33.82% of oxygen-containing groups in the interlayer reduce the amount of possible positions for Na + storage. After 1 h of thermal reduction, 23.80% of the oxygen-containing functional groups are removed, allowing more Na + to insert into the carbon interlayer of EG, despite the reduced interlayer distance of EG-1 h as 0.43 nm. EG-1 h can deliver a high reversible Na + capacity of ~300 mAh g −1 , which is significantly higher than PG and GO. When the reduction time extends to 5 h, the capacity of EG-5 h drops to ~100 mAh g −1 . Although similar charge–discharge pattern was observed between EG-1 h and EG-5 h, the capacity delivered by EG-5 h decreased significantly, implying that the interlayer distance predominantly controls the Na + storage capacity. The sodiation curve of EGs clearly consists of two stages, that is, monotonic sloping voltage profile between 2.0 and 0.3 V (versus Na/Na + ) and an inclined voltage plateau from 0.3 to 0.0 V (versus Na/Na + ). As reported by previous studies on Na storage in hard carbon and soft carbon, the monotonic curves occurring in the high voltage region (>0.3 V) correspond to insertion/extraction of Na + between graphene layers in EG [5] , [29] , whereas the low-voltage plateau may represent the Na + insertion/extraction in the pores/defects [5] , [29] . The slope in the low-voltage region (<0.3 V) in desodiation curve could be possibly attributed to hysteresis cause by the interaction between Na + and the residual hydrogen [5] , [30] . The second stage between 0.3–0.7 V should be corresponded to the Na + removal from pores, while the slope at high voltage range (>0.7 V) should be attributed to Na + extraction from graphitic layers. 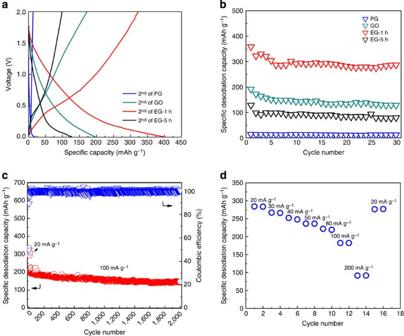Figure 5: Electrochemical performances. (a) Charge/discharge curves for the second cycles of PG, GO, EG-1 h and EG-5 h at a current density of 20 mA g−1. (b) Short-term cycling stability test for PG, GO, EG-1 h and EG-5 h at a current density of 20 mA g−1. (c) Long-term cycling stability of EG-1 h. Note that 20 mA g−1was used for the initial 10 cycles. At the 11th cycle, the current was changed to 100 mA g−1and held constant during the rest of the test. (d) Rate capability test for EG-1 h. Note that the cell was pre-cycled at 20 mA g−1for 20 cycles before the rate performance test. Capacities shown inb–dare specific desodiation capacities. Figure 5: Electrochemical performances. ( a ) Charge/discharge curves for the second cycles of PG, GO, EG-1 h and EG-5 h at a current density of 20 mA g −1 . ( b ) Short-term cycling stability test for PG, GO, EG-1 h and EG-5 h at a current density of 20 mA g −1 . ( c ) Long-term cycling stability of EG-1 h. Note that 20 mA g −1 was used for the initial 10 cycles. At the 11th cycle, the current was changed to 100 mA g −1 and held constant during the rest of the test. ( d ) Rate capability test for EG-1 h. Note that the cell was pre-cycled at 20 mA g −1 for 20 cycles before the rate performance test. Capacities shown in b – d are specific desodiation capacities. Full size image The EG has long range graphene layer stacked approximately parallel to each other producing relative turbostratic disorder, which is similar to soft carbon [5] . When Na-ion inserts into turbostratically arranged layers, the distribution of sites generates a range of chemical environments, thus a sloping potential curves [5] . However, when the sodium inserts into pores in the EG generated during oxidation/reduction process, there is very little charge transfer from the carbon to the sodium. Therefore, the sodium insertion into/extraction from pores shows a low-voltage plateau [5] . In addition, the existing of oxygen-containing groups such as –C=O could also contribute to Na + storage, exhibiting sloping profile at a high voltage range [31] . As an observed result, charge/discharge capacity initially increases (from PG, GO to EG-1 h), and then decreases (from EG-1 h to EG-5 h) with oxidation and reduction process. The cycling tests of PG, GO, EG-1 h and EG-5 h are shown in Fig. 5b . All materials show stable cycling performances in the first 30 cycles except the initial few cycles, with EG-1 h exhibiting the highest sodium storage capacity. So, EG-1 h was selected for further electrochemical tests and investigation of sodium storage mechanisms. And thus the term ‘EG’ that appears in the following sections refers to EG-1 h. Electrochemical performances of EG The long-term cycling stability of EG was investigated at a low cycling rate of 20 mA g −1 for the first 10 cycles to achieve a full sodiation capacity and then at a high current density of 100 mA g −1 , as shown in Fig. 5c . EG provides a capacity of ~280 mAh g −1 at 20 mA g −1 and ~180 mAh g −1 at a high current density of 100 mA g −1 . The EG demonstrates excellent cycling stability for 2,000 cycles with a very low capacity decay rate of ~0.013% per cycle from the 11th cycle to 2,000th cycle. Even though the sodium storage capacity of EG is similar to the reported soft carbon [5] and hard carbon [7] , [8] , the capacity retention of EG is much better. The first cycle coulombic efficiency of EG was ~49.53%, and approached 100% after ~10 cycles. Such a low first cycle coulombic efficiency was also reported for sodium storage in hard carbons (~40–60%; refs 7 , 8 ), and it was usually attributed to the formation of solid electrolyte interphase film, which can likely be reduced by (1) changing the electrolyte composition and (2) reducing the defects and voids of EG, both of which have been successfully applied to LIBs. For the rate capability tests, technologically significant capacities were achieved up to a current density of 200 mA g −1 . The specific cell was firstly cycled at 20 mA g −1 for 20 cycles to achieve stable cycling status before the rate capability experiment. As shown in Fig. 5d , EG exhibits a capacity of 284 mAh g −1 at 20 mA g −1 ; 184 mAh g −1 at 100 mA g −1 ; 91 mAh g −1 at 200 mA g −1 ; and 278 mAh g −1 when the current density is changed back to 20 mA g −1 , demonstrating the stability of EG under a wide range of charge–discharge conditions. The rate capability of EG is modest compared with reported hard carbon [8] , and it could be further improved through nanoengineering to optimize EG’s microstructure. Investigation on the sodium storage mechanism in EG Cyclic voltammetry was used to analyse the sodium storage mechanism. EG was tested at the scan rates of 0.05, 0.1, 0.5, 1, 2, 3, 5, 10 and 20 mV s −1 , as shown in Supplementary Fig. 6a . In Supplementary Fig. 6b,c , a linear relationship was found between the capacity and the reciprocal square root of scan rate, suggesting that the capacity was mainly limited by ion diffusion, similar to most battery electrodes [32] , because capacitive contribution, that is, pseudocapacitance because of surface reaction between Na + and oxygen-containing functional groups (for example, –C=O) [31] and double layer charging should be independent of the scan rate [33] . The capacitive contribution was approximately estimated by extrapolating the plot to V −1/2 QUOTE , and it only contributed to 10% of the total sodiation capacity ( Supplementary Fig. 6a ) and 11% of the total desodiation capacity ( Supplementary Fig. 6b ) at 0.05 mV s −1 (~0.1 C rate), indicating that the majority of the capacity is due to intercalation and it is highly reversible. This mixed storage mechanism was also observed for lithium storage in soft carbon [34] in which the lithium storage capacity from intercalation was found to be reversible and stable with cycling [34] . This explains the long and stable cycling performance of EG ( Fig. 5c ), as majority of the sodium storage capacity in EG is attributed to intercalation as demonstrated by Supplementary Fig. 6b,c . In situ TEM observation was conducted to provide further insights into the sodium storage mechanism and visualize microstructure evolution of EG during the sodiation and desodiation processes. 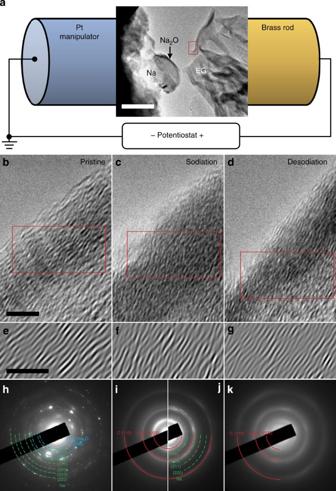Figure 6:In situTEM investigation of sodium storage mechanism in EG-1 h. (a) Schematic illustration of thein situexperimental setup. TEM graph shows EG-1 h on brass rod as the working electrode, Na metal on Pt manipulator as the counter electrode, and Na2O on Na surface as the solid electrolyte. Scale bar, 200 nm. The boxed region inacorresponds to high-resolution images inb–d. Typical microstructures of (b) pristine EG-1 h, (c) EG-1 h after the first sodiation, and (d) EG-1 h after the first desodiation. Scale bar, 5 nm. (e–g) Filtered TEM close-up images indicating representative microstructural features corresponding to the boxed areas inb–d, respectively. Scale bar, 5 nm. Electron diffraction patterns from (h) Na source area, (i) EG-1 h at pristine state, (j) EG-1 h after the first sodiation, and (k) EG-1 h after the first desodiation. Figure 6a illustrates the experimental setup of the NIB in the half-cell configuration, in which the EG glued on a brass rod with conducting adhesive serves as the working electrode, and the Na metal on a Pt manipulator as the counter electrode. A layer of naturally formed Na 2 O on the surface of Na source because of residual oxygen in the TEM vacuum is confirmed by the electron diffraction pattern from this area ( Fig. 6h ) and serves as the solid electrolyte for Na-ion transportation. The red boxed region at the curled edge of the graphite bulk was selected for high-resolution observations during the electrochemical reactions, and the corresponding close-up TEM morphologies for pristine EG, sodiated EG and desodiated EG are shown in Fig. 6b–d , respectively. To extract the relevant contrast, boxed areas at the approximate positions are re-plotted to display the representative features after filtering out high-frequency noise, as shown below the corresponding TEM images in Fig. 6e–g , respectively. The pristine EG displays a microstructure with well-aligned and long-range-ordered graphite layers ( Fig. 6b,e ) and contains large-scale pure graphitic structure with large interlayer distance ( Fig. 6i ). After contacting the surface Na 2 O electrolyte to the EG and applying a negative voltage of −3 V on the EG electrode (versus Na metal), the sodiation process initiates. As the Na ions migrate into the EG, the shape of the EG changes by tilting or distorting to accommodate the large-scale morphology changes. It is obvious that the microstructural disorder is complicated and more ripple-like features appear in the graphite-layered pattern ( Fig. 6c,f ). The electron diffraction pattern taken after the first sodiation ( Fig. 6j ) indicates that an amount of Na + has been accommodated into the EG. The sodiation-induced structure change was also observed by ex situ Raman spectra ( Supplementary Fig. 7 ). Compared with pristine EG, the intensity ratio between D band and G band becomes more pronounced for sodiated EG, indicating the increment in structure randomness after sodiation. Figure 6: In situ TEM investigation of sodium storage mechanism in EG-1 h. ( a ) Schematic illustration of the in situ experimental setup. TEM graph shows EG-1 h on brass rod as the working electrode, Na metal on Pt manipulator as the counter electrode, and Na 2 O on Na surface as the solid electrolyte. Scale bar, 200 nm. The boxed region in a corresponds to high-resolution images in b – d . Typical microstructures of ( b ) pristine EG-1 h, ( c ) EG-1 h after the first sodiation, and ( d ) EG-1 h after the first desodiation. Scale bar, 5 nm. ( e – g ) Filtered TEM close-up images indicating representative microstructural features corresponding to the boxed areas in b – d , respectively. Scale bar, 5 nm. Electron diffraction patterns from ( h ) Na source area, ( i ) EG-1 h at pristine state, ( j ) EG-1 h after the first sodiation, and ( k ) EG-1 h after the first desodiation. Full size image When a positive voltage is applied on the EG against the Na electrode, the desodiation process begins. As Na ions migrate out of the EG anode, the microstructure of desodiated EG is reversibly recovered to a parallel layered pattern with long-range ordering ( Fig. 6d,g ), and the residual Na ions in EG are found to be negligible as demonstrated by the disappearance of diffraction spots in Fig. 6k . It is also noted that, regardless of microstructural reorganization, the layered structure of the material does not exhibit large-scale distortion throughout the entire reaction, which provides a constant transport space for Na ions. Although the clear reaction front of these electrochemical reactions was not directly imaged, owing to insufficient volume change, the actual microstructural distortion and restoration associated with the sodiation and desodiation processes have been readily captured by in situ TEM. It is of great importance that such microstructural evolutions are reversible and reproducible without any mechanical or electrochemical breakdown for the observed six charge/discharge cycles ( Supplementary Fig. 8 , and would also be expected for further cycles according to the excellent cycling performance). Evident from the in situ TEM results, EG as the NIB anode material exhibits excellent performance attributed to the advantages of the unique and robust long-range layered structures. The in situ TEM results are consistent with post-mortem HRTEM study of after-cycled EG assembled in coin cells using liquid electrolyte. As shown in the HRTEM image in Supplementary Fig. 9 , after 150 sodiation–desodiation cycles, the EG still exhibits a long-lived layered structure with interlayer distance remaining at 0.42 nm, whereas the other local disordered contrast could be caused by effects of interaction with Na + morphologies. We have successfully developed EG with a long-range-ordered layered structure for NIB anodes. Different from other carbonaceous NIB anodes, EG stores Na + mostly by interlayer intercalation, which has been confirmed by cyclic voltammetry and in situ TEM observations through reversible interlayer expansion/shrinkage of the EG material during the sodiation and desodiation. The robustness of the long-range-ordered layered structure of EG during sodiation/desodiation has also been revealed by reproducible interlayer changes during multiple charge/discharge processes during in situ TEM observation. For practical NIB applications, EG can deliver a high reversible capacity of 284 mA g −1 at a current density of 20 mA g −1 , with superior capacity retention (73.92% after 2,000 cycles at 100 mA g −1 ). The findings reported here are beneficial for the design and manufacture of rechargeable sodium-ion batteries, positioning EG as a promising anodic material. GO and EG synthesis GO was synthesized through a modified Hummer’s method [13] . At room temperature, 1 g of graphite (synthetic, Sigma-Aldrich) and 0.5 g of NaNO 3 (reagent plus, Sigma-Aldrich) were added into 23 ml concentrated sulphuric acid (95–98%, ACS reagent, Sigma-Aldrich) in a round-bottomed flask. The flask was then put into an ice bath. Three grams of KMnO 4 (ACS reagent, Sigma-Aldrich) was added into the mixture slowly while stirring, during which the temperature was well controlled to lower than 20 °C. Then the temperature was brought to 35 °C and maintained for 2 h. Forty-six millilitres of room temperature H 2 O was added into the mixture slowly. The temperature was well controlled to below 98 °C during this process. After mixing, the temperature was then slowly brought up to 98 °C and maintained for 30 min. A quantity of 140 ml of warm water was further added to the liquid, followed by 20 ml of H 2 O 2 (30 wt% in H 2 O, Sigma-Aldrich), upon which golden particles and dark brown solid particles were formed. The mixture was filtered while still warm. Around 1 litre of warm H 2 O was further used to wash the solid until the supernatant was pH neutral at the end of washing. The resulting dark brown solid was collected as the GO product. To synthesize EG, the fore-mentioned GO was reduced by heat treatment. GO powder was put into alumina combustion boat in tube furnace with a continuous flow of Ar. The temperature was then brought from 25 to 600 °C with a heating rate of 5 °C min −1 . Then, the temperature was maintained at 600 °C for 1 and 5 h to reach different degrees of reduction. Material characterization The morphologies and microstructures of PG, GO and EG were characterized by a JEOL JEM-2100F TEM operated at 200 kV. For general structural characterization, the graphitic materials were transferred onto copper grids with amorphous carbon film support after stirring in isopropanol. For the XRD tests ( Supplementary Fig. 1 ), the sample was scanned from 5° to 90° at a scan rate of 0.5° per second in non-spin mode. The XRD data were collected by a D8 Advance diffractometer with LynxEye and SolX detectors in the X-ray Crystallographic Center at the University of Maryland. Brunauer–Emmett–Teller test was carried out on the Tristar II 3020 surface analysis system. In a typical measurement, ~100 mg of the powder sample was first degased for 5 h, and then loaded to the system for measurement. In a typical tap density test, ~1 g of the sample was put into a graduated measuring cylinder and then tapped for 50 times until no further volume change was observed. The volume was obtained by reading the inner diameter of the cylinder. The electronic conductivity of the samples was measured by four-probe method. In a typical measurement, powder sample with ~0.1 g in mass was assembled in a Swagelok cell with an inner diameter of 13 mm. The assembled cell was then loaded for 50 Mpa pressure for 3 min to achieve the pallets. The pallet samples were then measured using a four-probe method (Signatone SP4) at University of Maryland Nanocenter. Typical Raman tests ( Supplementary Fig. 2c ) were carried out over the dried powder samples. For the ex situ Raman characterization ( Supplementary Fig. 7 ), in a typical procedure, EG was assembled into a home-made glass cell with airtight structure. The cell was assembled with an EG working electrode, a sodium metal counter electrode and 1.0 M NaClO 4 in polycarbonate solvent liquid electrolyte in glove box with Ar atmosphere. Raman data were collected by Horiba–Jobin–Yvon Raman microscope in the University of Maryland Nanocenter with laser wavelength of 532 nm. XPS investigation was performed on powdered samples at room temperature. Data were collected using a high-sensitivity Kratos AXIS 165 spectrometer with survey pass energy of 160 eV and high-resolution pass energy of 20 eV, also at the University of Maryland Nanocenter. The solid-state NMR experiments were performed at 1 H frequencies of 500.16 MHz with Bruker Avance III system using a Bruker 3.2-mm triple-resonance E-free MAS probe in a double resonance mode. 13 C MAS spectra in Fig. 4 were collected by a rotor-synchronous echo sequence with ( Fig. 4a ) and without ( Fig. 4b,c ) a background suppression pulse sequence [35] using a Kel-F cap. The background suppression sequence was used in Fig. 4b,c to quantify the signals of very limited oxidized species without the effects of background signals. In the 13 C– 1 H REDOR experiments [36] , [37] , the data were collected with 13 C π-pulse sandwiched by 13 C– 1 H dephasing periods of four rotor cycles ( τ R =66.7 μs). The details are described in the Supplementary Material . Electrochemical characterization Electrochemical properties were characterized using a half-cell against a pure Na counter electrode. To assemble a test cell, the EG powder was mixed with 15 wt % of Na alginate in water in mortar and milled for 30 min. The resulting slurry was then cast on copper foil. After drying at room temperature for ~12 h, the sample was then transferred into a standard vacuum oven kept at 100 °C for overnight. A 0.5-inch circular die-punch was used to cut the electrode. The typical loading amount of active material was ~0.5 mg cm −2 . Coin cells, consisting of an EG electrode, a sodium metal counter electrode, Celgard 3501 separator and 1.0 M NaClO 4 in polycarbonate solvent liquid electrolyte, were assembled in a glove box under Ar atmosphere for further electrochemical tests. Galvanostatic charge/discharge was carried out on an Arbin BT-2000 test station. Cells were cycled between 0.0 and 2.0 V (versus Na/Na + ) at different current densities. After the cell reached the cutoff voltage, it was relaxed for 10 min before subsequent charge or discharge. The capacity was calculated based on the mass of active material. For the rate capability tests, cells were pre-cycled for 20 cycles for activation and then charged–discharged at different current densities between 0.0 and 2.0 V (Na/Na + ). The capacity is calculated based on the mass of EG. The cyclic voltammetry test was carried out on the Solartron 1260/1287 Electrochemical Interface test station (Solartron Metrology, UK). Cells were pre-cycled for 20 cycles to achieve the stable status before loaded to the testing system. The scan range was 0–2 V (versus Na/Na + ) with various scan rates. HRTEM characterization TEM characterization and in situ imaging were carried out on a JEOL 2100F transmission electron microscope operated at 200 kV. Regular HRTEM observation was conducted for ex situ samples to determine their structures and morphologies at different conditions. In situ HRTEM experiments were performed with a customized NanoFactory manipulation holder equipped with a piezo-driven Pt probe. The setup is shown in Fig. 6a . In a typical experiment, EG was glued onto a specimen rod using conductive Ag epoxy, and Na metal was scratched off a fresh-cut surface of Na bulk using the Pt manipulator inside a glove box filled with high-purity nitrogen to prevent oxidation. Then the Na metal was intentionally exposed to the air for <5 s during the holder loading process, in order to form a thin layer of Na 2 O on the surface, serving as a solid electrolyte. During the in situ operation, potentials of −1.0 V to −4.0 V were applied to EG with respect to Na metal to initiate sodiation, and +1.0 V to +4.0 V for desodiation. How to cite this article: Wen, Y. et al. Expanded graphite as superior anode for sodium-ion batteries. Nat. Commun. 5:4033 doi: 10.1038/ncomms5033 (2014).